Fully inorganic oxide-in-oxide ultraviolet nanocrystal light emitting devices The development of integrated photonics and lab-on-a-chip platforms for environmental and biomedical diagnostics demands ultraviolet electroluminescent materials with high mechanical, chemical and environmental stability and almost complete compatibility with existing silicon technology. Here we report the realization of fully inorganic ultraviolet light-emitting diodes emitting at 390 nm with a maximum external quantum efficiency of ~0.3%, based on SnO 2 nanoparticles embedded in SiO 2 thin films obtained from a solution-processed method. The fabrication involves a single deposition step onto a silicon wafer followed by a thermal treatment in a controlled atmosphere. The fully inorganic architecture ensures superior mechanical robustness and optimal chemical stability in organic solvents and aqueous solutions. The versatility of the fabrication process broadens the possibility of optimizing this strategy and extending it to other nanostructured systems for designed applications, such as active components of wearable health monitors or biomedical devices. The future development of numerous technological areas, from solid-state lightning and integrated photonics to sensors, relies on the realization of new light-emitting structures based on inexpensive, easily-workable and chemically stable materials. Over the last few years, a variety of solution-based synthesis methods have become available for producing high quality nanocrystals (NCs), either as self-standing colloidal nanoparticles [1] , [2] , [3] or as highly controlled crystalline nanophases in suitable host matrices [4] , [5] , [6] , [7] , thus combining the superior resistance of inorganic emitters over organic dyes to degradation with the advantages of inexpensive and large-scale fabrication processes, such as spin coating, contact and ink jet printing and layer-by-layer deposition [8] , [9] , [10] , [11] . Several examples of light-emitting diodes (LEDs) based on nanostructured (NS) materials have been reported by different groups [11] , [12] , [13] , [14] , and have shown a remarkable tunability across the visible spectrum [8] , [15] , [16] , [17] , [18] . The extension of the emission into the ultraviolet (UV) region is problematic and increasing efforts are being devoted to this task because of the technological relevance of UV-emitting solution processable nanomaterials [13] , [17] , [18] , [19] , [20] . The achievement of robust UV electroluminescent devices with reasonable electroluminescence (EL) efficiency remains, however, a long-standing goal in this field of materials research [14] , [19] , [20] , [21] , [22] . Potential applications include the integration of UV-LEDs on silicon chips for selectively triggering biological responses through site-specific UV irradiation or, when implemented in stretchable forms, the realization of UV-emitting structures for wearable biomedical devices, as successfully shown for red-emitting epitaxial AlInGaP quantum well structures on GaAs substrates [23] , [24] . Furthermore, UV-LEDs are widely applied to phosphor-based white LEDs, in which UV excitation ensures improved quality of 'warm' white light over systems pumped by blue LEDs [25] . In this framework, tin dioxide—with a direct forbidden optical gap of about 3.6 eV—has been demonstrated to be particularly suitable for producing wide-band-gap NSs in optical grade materials. SnO 2 NCs have been successfully obtained in transparent silica glass [5] , [26] with interesting optical properties, such as strong nonlinear response [27] , photosensitivity [28] and sensitized emission from rare-earth (RE) dopants excited via energy-transfer from the NCs [29] , [30] , [31] . Most relevant for this discussion, band-edge excitonic emission at 320–360 nm (refs 6 , 32 , 33 ) and radiative recombination mediated by shallow traps emitting at 370–390 nm (ref. 33 ) have been observed for a variety of SnO 2 nanostructures, such as colloidal suspensions [32] , nanowires [33] , NC films [34] , NCs embedded in silica by ion implantation [35] and thermally grown nanophase by selective nucleation of the molecular precursors in sol–gel silica [36] . The latter synthesis strategy opened the way to a possible design of robust UV-emitting structures based on NS SnO 2 :SiO 2 films spin-coated on silicon substrate, with benefits derived from a solution-based method, a full compatibility with existing silicon technology, and superior environmental stability resulting from the full inorganic architecture and the incorporation of the chromophores in silica. However, no report is present in the literature on LEDs based on such a material system. Tin oxides exhibit charge carriers with opposite signs depending on tin oxidation state and, ultimately, on tin coordination number. Specifically, SnO (litharge-like structure) is an intrinsic p-type semiconductor ( E gap =2.7–3.4 eV) with fourfold coordinated tin cations [37] , whereas SnO 2 (rutile-like structure) is an intrinsic n-type semiconductor with sixfold coordinated tin cations [38] . Nevertheless, one of the main drawbacks of tin oxides semiconductors lies in the spontaneous oxidation of Sn(II) to Sn(IV) when it is in contact with air. Therefore, in p-type SnO thin film transistors, inert oxide films such as SiO x or Al 2 O x are usually deposited as capping layers in order to preserve the tin oxidation state [39] , [40] . In this regard, the sol–gel nanoclustering approach is a suitable choice for the realization of efficient SnO 2 -based UV-LEDs for, at least, two reasons. First, tin atoms at the NC/matrix interfaces are expected to substitute silicon atoms in the tetrahedrally coordinated amorphous network, thus favouring the formation of fourfold coordinated tin oxide [36] . Second, once the sintering process is completed, the inert silica matrix protects the SnO x <2 NC shell against further oxidation by environmental agents. Recent investigations of the electric transport properties of SnO 2 :SiO 2 NS glasses revealed the crucial role of the under stoichiometric NC shell and interparticle distance on the percolative charge transport activated in the system [41] . Specifically, SnO 2 :SiO 2 NS systems with narrow interparticle distributions and NCs surrounded by thin under-stoichiometric SnO x <2 shells were found to be able to sustain both electron and hole currents under direct bias without charge accumulation in the nanophase that is usually associated with broad NC size dispersions [41] . Here we report the realization of ultraviolet LEDs based on NS SnO 2 :SiO 2 thin films from sol–gel synthesis. The concept of solution-processed NS UV-LEDs and their potential applications are summarized in Fig. 1 . Importantly, at variance with previously reported EL materials incorporating NCs from solution-processed methods, the fully inorganic architecture (without any organic layer), according to a fabrication protocol, which is suitable for the production of large area devices, ensures superior mechanical and chemical stability with a single deposition process. Furthermore, differently from other SnO 2 -based light-emitting hetero-junctions [42] , [43] , [44] , NCs with n-type cores and under-stoichiometric p-type shells provide a simultaneous flow of negative and positive charges that may radiatively recombine inside the NCs. 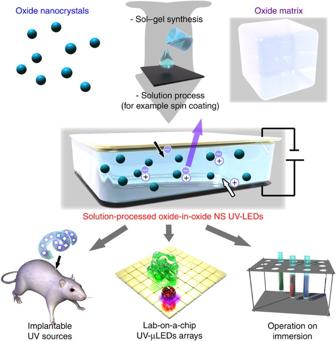Figure 1: Concept of solution-based oxide-in-oxide nanostructured LEDs and potential applications. The rational combination of wide-band-gap semiconductor oxide NCs with an insulating, transparent and chemically inert oxide matrix in a single-step fabrication process allows for the fabrication of robust ultraviolet (UV) electroluminescent materials capable, in principle, of operating in extreme conditions. The resulting nanostructured material features the chemical and physical properties of the NCs (such as nanocrystallinity, stoichiometry doping through metal/oxygen vacancies, chemical stability, wide-band-gap, ultraviolet emission) and the silica host (such as chemical stability, workability, compatibility with silicon and high transmittance in the ultraviolet spectral region). The lower panel displays some potential applications of oxide-in-oxide ultraviolet LEDs, achievable thanks to the full protection of the NC by the silica matrix. This type of solution-processed UV-LEDs may, in principle, be used in low-cost biomedical implants or micro/nano-patterned lab-on-a-chip platforms for biomedical diagnostics and environmental analysis under full immersion in aqueous or organic liquids. Figure 1: Concept of solution-based oxide-in-oxide nanostructured LEDs and potential applications. The rational combination of wide-band-gap semiconductor oxide NCs with an insulating, transparent and chemically inert oxide matrix in a single-step fabrication process allows for the fabrication of robust ultraviolet (UV) electroluminescent materials capable, in principle, of operating in extreme conditions. The resulting nanostructured material features the chemical and physical properties of the NCs (such as nanocrystallinity, stoichiometry doping through metal/oxygen vacancies, chemical stability, wide-band-gap, ultraviolet emission) and the silica host (such as chemical stability, workability, compatibility with silicon and high transmittance in the ultraviolet spectral region). The lower panel displays some potential applications of oxide-in-oxide ultraviolet LEDs, achievable thanks to the full protection of the NC by the silica matrix. This type of solution-processed UV-LEDs may, in principle, be used in low-cost biomedical implants or micro/nano-patterned lab-on-a-chip platforms for biomedical diagnostics and environmental analysis under full immersion in aqueous or organic liquids. Full size image The main obstacle for obtaining EL devices based on a tin–silicon oxide-in-oxide system is the low conductivity of the insulating silica-based matrix and the poor or null charge-injection features of the substrate interface that may undergo full oxidation during the thermal treatments of silica densification and NC growth. In the present work, we have tackled these problems by following four converging strategies. First, we designed and synthesized NS oxide-in-oxide films where the whole material acts as a distributed p – n junction where both hole and electron transport may take place in the device and, simultaneously, detrimental capacitive behaviours are minimized. Second, we minimized the NCs size in order to enhance possible quantum confinement effects and maximize the total passivated area at the NC/matrix boundaries. Third, we controlled the substrate oxidation, so as to obtain a SiO x layer between silicon and the NS film capable of sustaining charge injection [41] , [45] and, finally, we favoured electron injection from the cathode by using a low-work-function metal. Material synthesis and optimization Device and material features of our approach are summarized in Fig. 2 . The details of the synthesis and material optimization route that lead to the optimized final material are reported in the Methods section and Supplementary Figs S1–S3 . A representative scanning transmission electron microscopy image is reported in Fig. 2a showing the cross-section of a planar structure of SiO 2 :SnO 2 film (about 0.6 μm thick) on p -silicon with a SiO x interlayer (about 100 nm thick, and x <1 from intensity analysis of high angle annular dark field images) grown at the substrate interface. In the image collected in dark field, one may observe the dense nanoarchitecture of SnO 2 NCs inside the film (about 3×10 18 cm −3 and ~5 nm in size, appearing as small white spots) that has been demonstrated to be able to sustain electric currents of several tens of milliamperes without any measurable structural damage [41] . 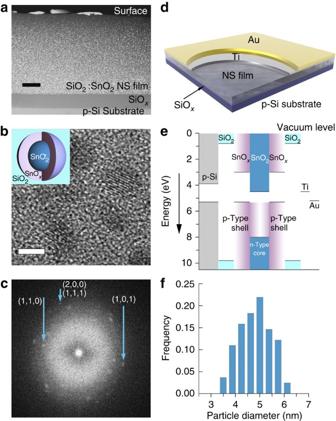Figure 2: Material and device structure. (a) Cross-sectional dark-field scanning transmission electron microscopy image of SiO2:SnO2NS glass ceramic film (~0.6 μm) grown on p-type silicon substrate, with a 100-nm thick SiOxinterlayer. Scale bar, 100 nm. (b) High-resolution transmission electron microscopy image of some SnO2nanocrystals. Scale bar, 4 nm. Inset: schematic representation of a NC structure showing the SnO2core (blue) surrounded by a substoichiometric SnOxshell (pink) in silica (cyan). (c) Fourier transform of previous image showing diffraction peaks belonging to SnO2in cassiterite crystal structure. (d) Schematic diagram of the device configuration of the ultraviolet nanostructured LED showing thep-silicon anode, the SiOxinterlayer, the NS SiO2:SnO2active layer, the semitransparent Ti anode (~5 nm) and the semitransparent gold capping layer (~10 nm). (e) Energy level scheme of the NS system showing the top level of the valence band and the bottom level of the conduction band in the SiO2matrix, in the SnO2NCs, and in the under-stoichiometric SnO-like interphase at the NC surface, as well as the band structure of p-Si substrate and the gate work function for Ti and Au electrodes (energy contributions from band bending, external electric field, Coulomb repulsion in charged NCs, and partially oxidized SiOxlayer are not included)41. The colour code for the different structural domains (NC core, shell and matrix) is the same as inb. (f) Statistical distribution of SnO2nanocrystal diameters. Figure 2b,c reports a representative high-resolution transmission electron microscopy image collected in bright field, as well as its Fourier transform, showing the typical size and crystalline features of the SnO 2 NCs. The schematic structure of the composite planar system is shown in Fig. 2d , including the p -silicon substrate and the semitransparent Au-capped titanium cathode (~10 nm Au; ~5 nm Ti). The choice of titanium as electrode assures a good electron injection into the conduction band of SnO 2 NCs ( Fig. 2e ), which favours electric conduction and the resulting generation of excitons inside the NCs. Furthermore, titanium ensures good adhesion on the glassy active film, which results in remarkably robust LEDs resistive to mechanical damage. Figure 2: Material and device structure. ( a ) Cross-sectional dark-field scanning transmission electron microscopy image of SiO 2 :SnO 2 NS glass ceramic film (~0.6 μm) grown on p-type silicon substrate, with a 100-nm thick SiO x interlayer. Scale bar, 100 nm. ( b ) High-resolution transmission electron microscopy image of some SnO 2 nanocrystals. Scale bar, 4 nm. Inset: schematic representation of a NC structure showing the SnO 2 core (blue) surrounded by a substoichiometric SnO x shell (pink) in silica (cyan). ( c ) Fourier transform of previous image showing diffraction peaks belonging to SnO 2 in cassiterite crystal structure. ( d ) Schematic diagram of the device configuration of the ultraviolet nanostructured LED showing the p -silicon anode, the SiO x interlayer, the NS SiO 2 :SnO 2 active layer, the semitransparent Ti anode (~5 nm) and the semitransparent gold capping layer (~10 nm). ( e ) Energy level scheme of the NS system showing the top level of the valence band and the bottom level of the conduction band in the SiO 2 matrix, in the SnO 2 NCs, and in the under-stoichiometric SnO-like interphase at the NC surface, as well as the band structure of p-Si substrate and the gate work function for Ti and Au electrodes (energy contributions from band bending, external electric field, Coulomb repulsion in charged NCs, and partially oxidized SiO x layer are not included) [41] . The colour code for the different structural domains (NC core, shell and matrix) is the same as in b . ( f ) Statistical distribution of SnO 2 nanocrystal diameters. Full size image The NC size distribution in a thin film annealed in controlled atmosphere of 2% oxygen in argon—suitable for limiting the oxidation of the substrate—is shown in Fig. 2f , with an average NC diameter of 4.8±0.7 nm. It is worth noting that this latter value is not intermediate between those observed in bulk samples sintered in vacuum and those in pure oxygen atmosphere (6.7 and 5.3 nm, respectively [41] ). Rather, the small crystallite sizes in the present samples turn out to be largely determined by the action of the chain terminators added in the sol (and absent in previous synthesis), in spite of the low oxygen pressure that has been observed to slightly increase the average NC size [41] . In fact, SnO 2 precipitation in SiO 2 occurs through a thermally activated nucleation in a supersaturated solid solution followed by a diffusion-limited crystal growth [5] . Hence, NCs precipitation may be controlled by the presence of heteroatoms or defects in the solid solution [26] . During crystal growth, these agents, could act both as pinning elements and diffusion inhibitors, leading to NCs size distributions centred at smaller mean diameters. Scanning electron microscopy images were also collected to control the morphology of the film surface and are reported in Fig. 3 . The optimization process indicated a treatment rate between 3 and 10 °C h −1 to avoid thermal shock and film fractures during the densification process. Some films showed the formation of micrometer-sized SnO 2 elongated crystals on the upper surface ( Fig. 3a ), drastically different from the homogenous surface of samples with lower SnO 2 content ( Figs 2a and 3b ). A detailed analysis of the possible causes indicated a correlation with the aging time of the tetramethoxysilane (TMOS) and dibutyltin diacetate (DBTDA) reagents. Large amounts of SnO 2 (~30% or higher) lead to substrate/film interfaces with weak adhesion properties, as confirmed by scanning electron microscopy analysis. Samples prepared with 40% of SnO 2 ( Fig. 3c–e ) clearly show poor adhesion and surface quality with cracked films. These evidences suggest that a large amount of NCs causes matrix stresses that may induce the mechanical instability responsible for the observed slashes and cracks. An extended discussion of the role of the sintering atmosphere and Sn concentration on the film morphology and adhesion properties is reported in the Methods section. 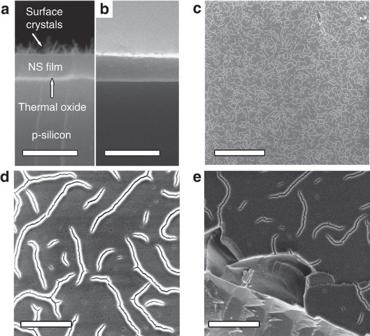Figure 3: Surface and adhesion analysis. (a) Scanning electron microscopy (SEM) image of a section of a nanostructured film on Si showing the formation of surface micrometer-sized crystals. (b) SEM image of the section of a NS film on Si annealed in oxidizing atmosphere. Scale bars inaandbcorrespond to 1 μm. (c–e) Representative SEM images of a NS film with poor adhesion properties and containing 40% SnO2, synthesized onp-silicon substrate. Scale bar inccorresponds to 100 μm, scale bars indandecorrespond to 10 μm. Figure 3: Surface and adhesion analysis. ( a ) Scanning electron microscopy (SEM) image of a section of a nanostructured film on Si showing the formation of surface micrometer-sized crystals. ( b ) SEM image of the section of a NS film on Si annealed in oxidizing atmosphere. Scale bars in a and b correspond to 1 μm. ( c – e ) Representative SEM images of a NS film with poor adhesion properties and containing 40% SnO 2 , synthesized on p -silicon substrate. Scale bar in c corresponds to 100 μm, scale bars in d and e correspond to 10 μm. Full size image We underlined that the proposed synthesis method is not limited to the production of NS films on silicon substrates, but is instead applicable to other thermally stable substrates such as quartz for producing transparent functional films on transparent media that can be further processed into waveguides or other optical patterns, thanks to the photorefractive response of the NS material [46] (Methods and Supplementary Fig. S4 ). The different energy gap of the NCs and the host, together with the chemical stability of the whole system, enable the use of a direct photo-writing process for the fabrication of refractive index patterns by exposure to focused laser beams. In NS SnO 2 :SiO 2 , laser pulses in the near-infrared, visible and near-UV spectral regions, are selectively absorbed by the NCs in the transparency region of the glass matrix through direct or multi-photon absorption processes [28] , [46] , [47] . As a result of the strongly localized energy release, partial amorphization of the nanophase takes place in the glass [28] , accompanied in some cases by local compaction of the surrounding host [46] . Nanophase amorphization and host compaction are concomitant mechanisms (tunable by changing the laser power density) that may be used to induce local permanent modification of the refractive index up to approximately ±10 −2 , either positive or negative depending on the process parameters [46] . Importantly, this type of top–down processing is entirely implementable to the proposed bottom–up strategy of material synthesis, thus allowing for the design of a wide class of optoelectronic devices. Since most of the current technologies are based on silicon, the feasibility of EL materials by wet chemistry approaches gains further relevance if compatible with silicon substrates. This feature may indeed provide a valid alternative to high-vacuum fabrication processes such as ion implantation or plasma-enhanced chemical vapour deposition, which have been used to fabricate silica-based emitting structures on silicon substrates [13] , [48] , [49] also in a view of their utilization as lab-on-a-chip diagnostic platforms [48] . Specifically, in this study, the choice of silicon as hole-injecting layer is made to demonstrate the feasibility of 'single block' solution-processed UV-LEDs where the substrate and the active layer become intimately connected in a new material system able to emit light as a result of transport mechanisms obtained through controlled synthesis conditions. 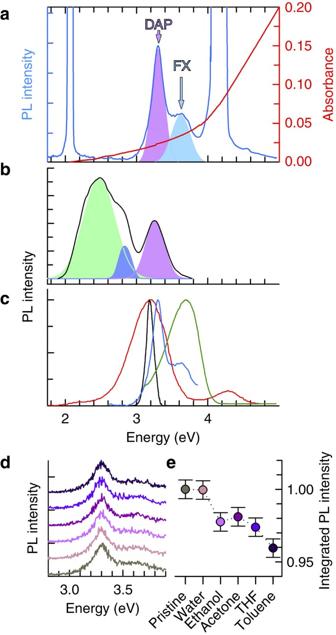Figure 4: Optical properties of nanostructured SnO2:SiO2films. (a) Photoluminescence (PL) spectrum (blue line) excited at 4.1 eV (300 nm), together with its Gaussian deconvolution, of a NS film grown on silicon substrate and absorption spectra (red line) collected for a film grown on transparent silica substrate. The PL spectrum shows two distinct contributions due to radiative recombination of SnO2free excitons at ~3.62 eV (FX, cyan band) and to radiative exciton recombination in donor–acceptor sites at ~3.3 eV (DAP, pink band36). (b) PL spectrum (black line) excited at 4.7 eV (266 nm) of the same NS film as inatogether with its Gaussian deconvolution, showing three contributions arising from: SnO2defects (green band at 2.5 eV, ref.52), silicon-related oxygen deficiency centres (ODCs, blue band at 2.8, ref.49) and DAP emission (pink band at 3.3 eV). (c) Comparison of the observed PL (blue line, same as ina) with the emission spectra of Sn-related ODCs (red curve49), colloidal SnO2NCs (green curve32) and exciton PL at donor–acceptor sites in SnO2nanowires (black curve50). (d) PL spectra excited at 4.1 eV of a NS film before (Pristine) and after immersion in several solvents (from bottom to top: Pristine, water, ethanol, acetone, THF, toluene). (e) Integrated PL intensity in the region 2.3–3.9 eV. All measurements have been conducted in the same condition of excitation fluence and detection geometry. The colour code is the same for panelsdande. Optical properties of NS films Figure 4 summarizes the main optical features of a NS thin film, showing the absorption spectrum of a film grown on a transparent substrate and the photoluminescence (PL) spectra of a film excited at 4.1 and 4.7 eV ( Fig. 4a,b , respectively). The absorption tail evidences the formation of a phase with E g ~3.6 eV consistent with SnO 2 nanoprecipitation. The PL spectrum excited at 4.1 eV shows two distinct contributions, both in the UV spectral region, due to radiative recombination of SnO 2 -free excitons at ~3.6 eV (FX, cyan band) and to radiative decay of excitons in donor–acceptor sites [33] , [50] at ~3.3 eV (pink band). Importantly, in this excitation condition, no emission from Sn-related oxygen deficiency centres (ODCs) [49] or SnO 2 defects in the visible spectral region is observed. In contrast, excitation at 4.7 eV ( Fig. 4b ) allows for direct excitation of both such defect sites, and therefore, the PL spectrum shows three main spectral features: the exciton-like emission peaked at ~3.3 eV (coloured in pink in analogy to the same emission observed at 4.1 eV excitation), a weak band at 2.8 eV, and a broad and intense emission at 2.5 eV arising from defect states due to silicon-related ODCs [49] and non-bridging oxygen centres of bulk SnO 2 (ref. 51 ), respectively. Figure 4: Optical properties of nanostructured SnO 2 :SiO 2 films. ( a ) Photoluminescence (PL) spectrum (blue line) excited at 4.1 eV (300 nm), together with its Gaussian deconvolution, of a NS film grown on silicon substrate and absorption spectra (red line) collected for a film grown on transparent silica substrate. The PL spectrum shows two distinct contributions due to radiative recombination of SnO 2 free excitons at ~3.62 eV (FX, cyan band) and to radiative exciton recombination in donor–acceptor sites at ~3.3 eV (DAP, pink band [36] ). ( b ) PL spectrum (black line) excited at 4.7 eV (266 nm) of the same NS film as in a together with its Gaussian deconvolution, showing three contributions arising from: SnO 2 defects (green band at 2.5 eV, ref. 52 ), silicon-related oxygen deficiency centres (ODCs, blue band at 2.8, ref. 49 ) and DAP emission (pink band at 3.3 eV). ( c ) Comparison of the observed PL (blue line, same as in a ) with the emission spectra of Sn-related ODCs (red curve [49] ), colloidal SnO 2 NCs (green curve [32] ) and exciton PL at donor–acceptor sites in SnO 2 nanowires (black curve [50] ). ( d ) PL spectra excited at 4.1 eV of a NS film before (Pristine) and after immersion in several solvents (from bottom to top: Pristine, water, ethanol, acetone, THF, toluene). ( e ) Integrated PL intensity in the region 2.3–3.9 eV. All measurements have been conducted in the same condition of excitation fluence and detection geometry. The colour code is the same for panels d and e . Full size image The ultraviolet band at 3.3 eV in SnO 2 observed under both 4.1 and 4.7 eV excitation may have two different origins: a well-known defect emission ascribed to tin-related ODCs in silica with a full-width at half-maximum (FWHM) of 0.57 eV (ref. 49 ) and the superposition of several contributions recently attributed to exciton bound to neutral donor (D 0 X) and donor–acceptor pair (DAP) recombinations [33] , [50] with a total FWHM of 0.13 eV. In regard to SnO 2 in low-dimensional systems, the strong quantum confinement causes the E g to shift towards higher energies and enables free-exciton decay (FX) [32] , [36] at 3.5–4 eV with a FWHM of 0.53 eV. Figure 4c displays the three possible UV emissions related to tin oxide compounds: Sn ODC in silica, DAP emission and FX radiative decay in quantum confined SnO 2 systems. Indeed, the UV PL emission observed in our films at 4.1 eV excitation, which is centred at 3.30 eV with FWHM=0.18 eV, has spectral features which evidently differ from the defect band, and are closer to those of DAP emission. We may consider this emission as an exciton-like one, although contributions of shallow donor/acceptor levels are likely involved. A crucial feature of our oxide-in-oxide systems is the enhanced chemical stability provided by the inert silica matrix, which shields the emitting sites from detrimental effects due to external agents. As a result, the optical properties of the NS material are unaffected by organic and/or aqueous solvents, thus making it suitable for application in direct contact with potential quenching agents. To provide a clear demonstration of this important property, we measured the PL response of a NS film excited at 4.1 eV after successive dipping in aqueous and organic solvents. The results reported in Fig. 4d,e show no change of both the spectral shape and the PL intensity, thus confirming the remarkable protection of the emitting sites achievable through the incorporation of NCs in the oxide matrix. Ultraviolet LED response Representative results achieved through the strategy described above for the fabrication of UV-LEDs based on SnO 2 NCs in silica are summarized in Fig. 5 . Ultraviolet EL spectra and electrical response of a layered structure with Sn content of ~16% are reported in Fig. 5a,b , respectively. The detailed discussion of the correlation between the structural properties of the NS film, controllable through different synthesis conditions and thermal annealing procedures, and the electric transport mechanism in both forward and reverse bias are reported in the Supplementary Discussion ( Supplementary Figs S5 and S6 ). 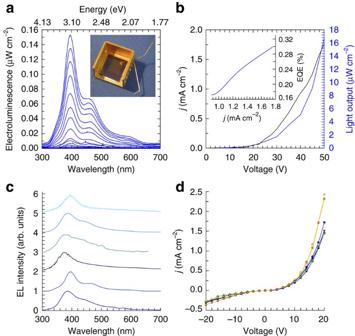Figure 5: Ultraviolet electroluminescence spectrum and electric response of NS-LEDs. (a) Electroluminescence spectrum of a NS-LED at increasing bias voltage. The active layer consists of a sol–gel silica matrix with SnO2NCs (nominal Sn concentration 16 mol%). The inset shows a photograph of a NS-LED (size: 2×2 cm2). (b) Current density and light output versus applied voltage of the ultraviolet NS-LED. Inset: external quantum efficiency (EQE), from the top face of the device, as a function of current densityj. (c) Electroluminescence spectra of six different NS-LEDs with undoped and Er3+-doped SnO2:SiO2active layers showing the reproducibility of the obtained results. Nominal Sn content and driving voltage from bottom to top: 15% Sn, 35 V; 16% Sn, 38 V; Er3+:15% Sn, 35 V; Er3+:15% Sn, 38 V; 18% Sn, 45 V; 15% Sn, 37 V. Erbium-doped films (0.3 mol%) show EL spectra peaked further in the ultraviolet with respect to the undoped material, in agreement with the smaller NC sizes observed in rare-earth-doped SnO2:SiO2systems26. (d) Electric response of an ultraviolet NS-LED (nominal Sn concentration 16 mol%) while immersed into several organic and inorganic solvents: water (dark blue triangles), ethanol (blue squares), acetone (green diamonds), THF (yellow triangles) and toluene (orange hexagons). Figure 5c reports the EL spectra under forward bias of six different NS-LEDs showing the reproducibility of the results. A photograph of a working NS-LED showing the visible portion of the EL emission is reported in Fig. 6 together with the EL spectrum and the optical response of the camera used to collect the photographs. Figure 5: Ultraviolet electroluminescence spectrum and electric response of NS-LEDs. ( a ) Electroluminescence spectrum of a NS-LED at increasing bias voltage. The active layer consists of a sol–gel silica matrix with SnO 2 NCs (nominal Sn concentration 16 mol%). The inset shows a photograph of a NS-LED (size: 2×2 cm 2 ). ( b ) Current density and light output versus applied voltage of the ultraviolet NS-LED. Inset: external quantum efficiency (EQE), from the top face of the device, as a function of current density j . ( c ) Electroluminescence spectra of six different NS-LEDs with undoped and Er 3+ -doped SnO 2 :SiO 2 active layers showing the reproducibility of the obtained results. Nominal Sn content and driving voltage from bottom to top: 15% Sn, 35 V; 16% Sn, 38 V; Er 3+ :15% Sn, 35 V; Er 3+ :15% Sn, 38 V; 18% Sn, 45 V; 15% Sn, 37 V. Erbium-doped films (0.3 mol%) show EL spectra peaked further in the ultraviolet with respect to the undoped material, in agreement with the smaller NC sizes observed in rare-earth-doped SnO 2 :SiO 2 systems [26] . ( d ) Electric response of an ultraviolet NS-LED (nominal Sn concentration 16 mol%) while immersed into several organic and inorganic solvents: water (dark blue triangles), ethanol (blue squares), acetone (green diamonds), THF (yellow triangles) and toluene (orange hexagons). 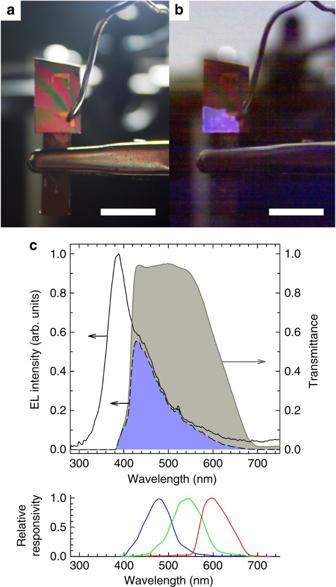Figure 6: Photographs of an ultraviolet NS-LED (15% Sn content) on ap-silicon substrate with Ti/Au cathode (5 nm Ti; 10 nm Au) at (a) 0 V and (b) 40 V applied bias (J=0. 4 mA cm−2). Homogeneous EL emission is observed from the whole device surface. Scale bars inaandbcorrespond to 10 mm. (c) Top panel: EL spectrum of the NS-LED (black solid line) and transmission spectrum of the standard optics of the photo camera (grey) used to collect the photographs inaandb. The visible portion of the EL emission detected by the camera is shown as a dashed line and shaded in purple. Bottom panel: normalized spectral responsivity of the red, green and blue (RGB) pixels of the camera. Importantly, the sensitivity of the camera is essentially zero below 400 nm, which further prevents to collect the main ultraviolet electroluminescence emitted by the NS-LED. Full size image Figure 6: Photographs of an ultraviolet NS-LED (15% Sn content) on a p -silicon substrate with Ti/Au cathode (5 nm Ti; 10 nm Au) at ( a ) 0 V and ( b ) 40 V applied bias ( J =0. 4 mA cm −2 ). Homogeneous EL emission is observed from the whole device surface. Scale bars in a and b correspond to 10 mm. ( c ) Top panel: EL spectrum of the NS-LED (black solid line) and transmission spectrum of the standard optics of the photo camera (grey) used to collect the photographs in a and b . The visible portion of the EL emission detected by the camera is shown as a dashed line and shaded in purple. Bottom panel: normalized spectral responsivity of the red, green and blue (RGB) pixels of the camera. Importantly, the sensitivity of the camera is essentially zero below 400 nm, which further prevents to collect the main ultraviolet electroluminescence emitted by the NS-LED. Full size image The ultraviolet EL spectra ( Fig. 5a ) are peaked at about 390 nm, with a light output of about 16 μW cm −2 at a current density of about 1.8 mA cm −2 ( Fig. 5b ) and remarkable maximum external quantum efficiency (EQE) of ~0.3%, which is comparable to recently reported efficient all-inorganic NC-LEDs emitting in the red spectral region (~0.1%) [12] . As already discussed for the PL emission, minor contributions in the EL spectra at 460 and 590 nm arise from radiative recombination of deep traps located at the NC/matrix interface and are attributed to ODCs and non-bridging oxygen centres, respectively [49] . Beside the minor presence of defect-related emission in the visible spectral region, the EL spectra resemble well the PL excited at 4.1 eV ( Fig. 4a ), which suggest that the exciton-like EL due to radiative recombination of electron-hole pairs close to the NCs band-edge is selectively excited by charge percolation through low-energy pathways, which is incapable of exciting SnO 2 or SiO 2 ODCs, as it is instead possible by using high-energy photons at 4.7 eV. It is noteworthy that similar electric response and EQE are registered for different devices, as shown in Fig. 5c . In this figure, two examples of erbium-doped SnO 2 :SiO 2 LEDs are also reported demonstrating the possibility of controlling the spectral emission by tuning the nanoarchitecture of the material. As already mentioned, in bulk samples, RE doping has been shown to shift the NC size distribution towards smaller sizes [26] , causing the band gap to widen. Concomitantly, RE ions passivate the substoichiometric NC/silica interface resulting in increased exciton emission [36] . Both these modifications are consistent with the specific and reproducible effects represented by the EL spectra of the two erbium-modified films in Fig. 5c . It is worth noting that NS-LEDs showed stable EL performances although they were tested in air over several days without additional environmental packaging, and were stored in atmospheric conditions between experiments. Importantly, our LED architecture does not include luminescent charge-injecting layers, which may excite the NCs via energy-transfer processes. Therefore, the observed EL is exclusively due to charge injection directly into the active layer. We note that the turn-on voltage of both current and EL (~20 V) is still relatively high compared to visible emitting NC-LEDs (~6–10 V). This is most likely due to the thickness of the SiO x interlayer and the NS film (~600 nm versus typical thicknesses of few close packed NC monolayers). Importantly, the EL emission is detected from the top face of the LEDs through the semi-transparent Ti/Au electrode (total thickness ~15 nm, transmittance at 390 nm ~30%). The reported EQE is not corrected for the losses due to reflection by the top electrode, and it represents the operative efficiency of our systems in the device configuration, which is the relevant parameter for application. At any rate, taking the losses due to reflection by the top electrode into account would lead to an internal efficiency over a factor of three higher than the measured EQE. Finally, in Fig. 5d , we report the electric response of the same device as in Fig. 5a while immersed into several organic and inorganic solvents: water, acetone, ethanol, toluene and tetrahydrofuran (THF). In agreement with the PL data in Fig. 4d,e , the electric response of the device is unaffected by the solvents. These results clearly demonstrate the effectiveness of the oxide-in-oxide architecture with a chemically inert silica matrix that ultimately confers to the whole NS material the chemical stability of silica glass while preserving the transport properties due to the controlled segregation of n-type NCs with substoichiometric p-type interfaces. In summary, we have demonstrated that purely inorganic ultraviolet LEDs with good emission yields (~0.3%) and light output performances can be fabricated by using UV-emitting NCs embedded in insulating SiO 2 films. As a result of the protection of the NCs ensured by the transparent glassy matrix, the reported UV-LEDs may in principle enable operation even during immersion in water or physiological solutions, hence, constituting active components of wearable health monitors or biomedical devices. The versatility of the fabrication process, which consists of an easily reproducible single-step solution-based synthesis, indicates the possibility of optimizing this strategy and extending it to other NS systems for designed applications. Material synthesis and sample preparation Ultraviolet-emitting devices with SnO 2 NCs embedded in SiO 2 films were fabricated by spin coating a solution of organic molecular precursors of silicon and tin on p -silicon wafers, followed by a thermal treatment during which organic residuals are removed, porosity collapses and SiO 2 network densification occurs, parallel to the thermally activated nanoclustering of tin dioxide [41] . A flux diagram of the synthetic route is reported in Supplementary Fig. S1 . The synthesis starts from a solution composed by TMOS and DBTDA in THF, with the addition of trimethylsilyl acetate (TMSA) and trimethyl methoxy silane (TMMS) to control the linking properties of the solution and to keep its viscosity at suitable values for spinning purposes without too high a dilution, which could greatly limit the desirable film thickness. Volume ratios THF/TMOS/TMSA/TMMS set to 7.5:1:0.125:0.075 were adopted. Tin doping with concentration in the range of 9–30 mol% (with respect of Si) was obtained through the addition of DBTDA to the mixture. The hydrolysis starts as pure water is added to the sol, with a volume ratio H 2 O/TMOS equal to 0.6:1. Before spin-coating, the sols were aged over times ranging from 124 h to 48 h, depending on the concentration of the tin molecular precursor, which has catalytic effect on the sol–gel reaction and requires early deposition for the more concentrated sols. In Sn-doped low-density SiO 2 films, the nucleation of the SnO 2 nanophase is thermally activated through a slow condensation treatment carried out by heating the samples from room temperature up to ~1,000 °C with a heating rate of 5 °C h −1 in the temperature range of 40–450 °C, and 10 °C h −1 in the 450–1,000 °C range. The first stage of the sintering process is held in a 0.3% vol oxygen/argon mixture, whereas the second one is carried out in a higher partial pressure oxygen set to 2% vol . RE nitrate was also added to produce RE doped films; Er precursor was used, obtaining 200–5,000 p.p.m. doping. The fabrication of inorganic glass-based NS films was designed after collecting detailed data on bulk materials about the possible strategies for chemically controlling the nanostructuring of sol–gel-derived inorganic glasses, specifically investigating the effects of co-doping with RE ions or fluorine precursors, as well as the effects of the oxygen partial pressure during thermally activated nanoclustering [26] , [52] , [53] . Sols were produced starting from TMOS, DBTDA in THF. Other solvents, silicon precursor and tin precursor are suitable as well (for example, tetraethyl orthosilicate, TEOS, for silica and molecules within the class R a Sn X b were R is an alkyl group and X is a hydrolysing group similar to alcoxide or acetate and a and b are stoichiometric coefficients with a suitable value). From the collected data, the investigation started by trying the best method for implementing the synthesis route for the production of films as layer-on-substrate systems. This target implied to overcome the problems related to nanostructuring homogeneity, adequate thickness to enable optical activity and enhanced electric conductivity for the charge transport into the final electrically driven device. Main parameters investigated in this step were the sol viscosity and the gelation rate. The results showed that in order to obtain thin films with thickness between 50 and 2,000 nm, the colloidal properties of the sol can be usefully modified by adding silicon compounds with hydrolysable and non-hydrolysable (as alkyl groups) ligands ( Supplementary Fig. S1 ). Molecules preferentially used to this purpose are: TMSA and TMMS. These chemicals act as 'chain terminators' and operate by reducing the networking and the colloid dimension. The effect on the sol properties is remarkable, and the concentration of the precursors can be controlled to achieve films of desired thickness. Typical sol compositions of glass ceramics films optimized through the analysis of the change of gelation rate within a wide range of starting concentration of reagents are exemplified in Supplementary Table S1 . In first example, RE nitrates or complexes were also added to produce RE-doped glass ceramics. Er, Ce, Eu precursors were used, obtaining 200–5,000 p.p.m. doping levels. Other metals can be added. After the 5 or 6 days in thermostatic chamber needed for the hydrolysis and condensation reactions to occur, the sols were deposited by the spin-coating technique. The obtained films were then sintered in controlled atmosphere. A typical thermal treatment starts at room temperature and ends at ~1,000 °C. As a result of the treatment, organic residuals are removed, porosity collapses, the network densifies and finally the phase segregation of tin (IV) oxide is successfully induced. Usually, a first stage between room temperature and 400 °C is kept under low partial pressure of oxygen (0.5–2% in inert gas) to avoid an excessive shock to the partially organic network of these films. At higher temperature, oxygen partial pressure can be changed to adjust the phase-separation parameters. The effects of changing the oxygen pressure were indeed investigated at the following values: 0.3, 2, 3.4% O 2 at different values of Sn concentration ( Supplementary Table S2 ). Thickness and refractive index of the films were measured after the thermal treatment by means of the prism coupler and m-lines methods. In Supplementary Figure S2 , the refractive index n and the film thickness d of a representative glass ceramic film (example 3 in Supplementary Table S1 ) are shown for three steps of the process, as they result from the analysis of the reported measurements of guided optical modes at 633 nm. Other representative data are reported in Supplementary Fig. S3 . The refractive index appears to depend mainly on the Sn content, which enhances the refractive index value as expected, but with noteworthy effects related to the treatment condition. Scanning electron microscopy images were also collected to control the morphology of the film surface. As shown in the SEM image in Supplementary Fig. S4 , a too high oxygen pressure causes the formation of a thick thermal oxide layer at the interface between substrate and deposited film. The optimization process indicated a treatment rate between 3 and 10 °C h −1 to avoid thermal shock and film fractures during the densification process. Some films showed the formation of micrometer-sized SnO 2 -elongated crystals on the upper surface ( Fig. 3a ). A detailed analysis of the possible causes indicated a correlation with the aging time of the TMOS and DBTDA reagents. Samples containing very high tin content (>30% mol) showed poor surface quality, as reported in Fig. 3b–d , because of mechanical stresses between matrix and SnO 2 NCs. At the end of the morphology optimization, homogeneous films were obtained, suitable for the deposition of metal gates. Before metal deposition, the material structure was checked by means of microFTIR spectroscopy in the spectral range 400–4,000 cm −1 . The results reported in Supplementary Figure S3 show the full condensation of the sol–gel matrix, with the formation of a densified silica glass embedding a SnO 2 phase. In fact, all the spectra show the typical contribution of Si–O–Si phonon modes at 450, 1,080, 1,240 cm −1 , attributed to rocking transverse optical (TO), and TO and longitudinal optical (LO) antisymmetric stretching, of Sn–O–Sn modes (just above 450 cm −1 and below 700 cm −1 ), besides other modes from the Si substrate at 460 cm −1 and in the region at around 648 cm −1 . At higher energy, above 1,500 cm −1 , there are mixed modes, overtones and modes due to hydroxyl groups. The differences from sample to sample in the modes at 1,080, 1,160 and 1,250 cm −1 (reflecting SiO 4 tetrahedra distortions and variations of the mean bond angle Si–O–Si) [54] are ascribable to different levels of structural disorder in the silica matrix, depending on the synthesis and treatment conditions [55] . Finally, semitransparent gold-capped titanium layers (5 nm Ti; 10 nm Au) are deposited by ion beam and thermal evaporation, respectively, on the resulting optimized NS films, about 600 nm thick, with the p -silicon wafer acting as lower electrode. Films on fused quartz substrate (2 cm in diameter and 0.5 mm thick) were prepared following the same synthesis route used for films on silicon substrates. Samples with nominal tin concentration of 9, 13 and 30%mol were sintered at 1,100 °C, heating rate 10 °C h −1 , in controlled atmosphere of 0.2% (low pO 2 ) or 3% (high pO 2 ) of oxygen in pure argon. Samples with 9 and 13% of SnO 2 were flat and homogenous with average surface roughness of ~50 nm as determined by profilometer analysis (Diktat 8 Veeco). In contrast, the surface of samples with 30% of SnO 2 showed irregularities with fragments indicating a partial exfoliation of the film. In Supplementary Fig. S4 , we report transmission spectra of pristine and cleaned films. Cleaning (with lens paper and acetone) removes the film containing 30% of SnO 2 and the spectrum is indistinguishable from the substrate. On the other hand, upon cleaning, samples with lower SnO 2 content show only a slight increase of transmittance. Optical transparency is maintained in the whole visible and near-infrared (NIR) regions and the presence of SnO 2 affects only the ultraviolet portion of the spectra. Sintering atmosphere gives some minor effects on the transmittance: it is lower in samples prepared in high partial pressure of oxygen. Material and device characterization Structure and morphology of the deposited material were respectively analysed by means of attenuated total reflection Fourier transform infrared spectroscopy—looking at the spectral features of the SiO 2 phonon modes at around 1,100 cm −1 , which are indicators of the matrix densification—and by scanning electron microscopy and transmission electron microscopy for controlled thickness and surface homogeneity, as well as material NS. Mean thickness and refractive index of the films were determined by the analysis of guided modes detected by means of a prism coupler refractometer operating at 633 nm. NS films were also deposited on transparent pure silica substrates to measure the absorption spectrum and to identify the SnO 2 nanophase band gap at about 3.6 eV. PL spectra were excited at 266 nm with the fourth harmonic of a pulsed Nd:YAG laser and at 300 nm with a filtered xenon lamp and collected with a phototube coupled with a single grating monochromator. Electroluminescence measurements were carried out by applying positive DC voltage to the p -silicon substrate. The emitted light was collected either by using a calibrated photodiode for measuring the integrated emission as a function of electric current, or by a photomultiplier tube coupled to a spectrometer for the spectral analysis of the EL emission. How to cite this article: Brovelli, S. et al . Fully inorganic oxide-in-oxide ultraviolet nanocrystal light-emitting devices. Nat. Commun. 3:690 doi: 10.1038/ncomms1683 (2012).